Diffraction using laser-driven broadband electron wave packets Directly monitoring atomic motion during a molecular transformation with atomic-scale spatio-temporal resolution is a frontier of ultrafast optical science and physical chemistry. Here we provide the foundation for a new imaging method, fixed-angle broadband laser-induced electron scattering, based on structural retrieval by direct one-dimensional Fourier transform of a photoelectron energy distribution observed along the polarization direction of an intense ultrafast light pulse. The approach exploits the scattering of a broadband wave packet created by strong-field tunnel ionization to self-interrogate the molecular structure with picometre spatial resolution and bond specificity. With its inherent femtosecond resolution, combining our technique with molecular alignment can, in principle, provide the basis for time-resolved tomography for multi-dimensional transient structural determination. Direct visualization of isolated molecules undergoing structural transformations can provide insight into the fundamental understanding of chemical processes [1] , [2] . Conventional methods based on diffraction and absorption [1] , [2] , [3] , [4] , using electrons or synchrotron-generated X-rays pulses, routinely achieve sub-angstrom resolutions, but their picosecond duration precludes characteristic, femtosecond-scale dynamical molecular imaging [4] , [5] , [6] , [7] , [8] . The recent development of femtosecond sources [9] , [10] of X-rays, for example, free-electron lasers, and electron beams has enhanced the temporal resolving power of these standard probes for ultrafast molecular dynamics [11] , [12] , [13] . Femtosecond electron and X-ray diffraction have been successfully demonstrated recently [14] , [15] , [16] , [17] . These schemes offer the potential for performing ultrafast dynamic imaging in condensed-phase systems, but their current fluxes are insufficient to achieve good enough signal-to-noise ratios for more rarified systems, for example gas-phase. Alternatively, since electrons have larger diffraction cross-sections than X-rays [1] , it is advantageous to convert X-ray photons to electrons via core ionization [18] , [19] , [20] . Femtosecond photoelectron diffraction/holography has been proposed as a time-resolved imaging method of transient molecules in the gas phase [21] , [22] . Since its advent, the intense ultrafast infrared laser pulse has been another enabling technology for time-resolved imaging on table-top systems. Combining conventional electron or X-ray beam methods with femtosecond laser pulses provides improved temporal resolutions for molecular dynamics investigation approaching atomic time scales [23] , [24] , [25] , [26] . However, recent experiments [27] , [28] , [29] , [30] , [31] demonstrated that intense, isolated femtosecond pulses alone are sufficient for imaging simple molecules via a strong-field three-step process [32] , [33] (see Supplementary Discussion ). First, the intense, low-frequency laser ionizes the molecule. Second, the continuum electron is accelerated in the laser field. Third, approximately three quarters of a laser period later, the high-energy electron revisits and elastically scatters off its parent ion. Conceptually this is analogous to the external electron beam used in conventional electron diffraction (CED) studies. Dubbed laser-induced electron diffraction (LIED) [34] , [35] , the method relies on extracting elastic differential cross-sections (DCS) from the two-dimensional (2D) photoelectron angular distributions [27] , [28] , [29] , [30] , [31] . Recently, picometre and femtosecond resolutions were demonstrated for N 2 and O 2 bond distance determination by fitting the extracted angle-dependent elastic DCS [36] . Here, we show a simpler approach that directly connects a femtosecond measurement to a simple 1D Fourier transform for determining atomic positions with picometre precision. Independent of the method, the critical parameter that ultimately controls the spatial resolution is the momentum transfer, | q |, defined as | q |=2| k r |sin( θ r /2), where k r and θ r are the electron’s scattering momentum and angle, respectively. In a typical CED experiment | k r | is held constant and | q | is varied by sweeping the angle, usually over a small range in the forward direction. However, similar | q | ranges can be obtained at a fixed angle (with the most advantageous collision geometry for θ r =180°) by varying the electron momentum. In strong field ionization, the backscattering requirement is met along the laser polarization, in which case the photoelectron energy distribution exhibits a long backscattering plateau [37] . The maximum detected electron energy extends to ~10 U P , where U P represents a free electron’s cycle-averaged quiver energy (called ponderomotive energy). This cutoff corresponds to a ~3 U P electron-ion recollision energy, which decreases monotonically for electrons detected at lower energies. The correspondence between detected and recollision electron energy is identical with LIED (see Supplementary Information in ref. 36 ). As a function of laser intensity I (10 14 W cm −2 ) and wavelength λ (μm), the ponderomotive energy is U P (eV)=9.3 Iλ 2 . For small molecules, it has been demonstrated that mid-infrared wavelengths ( λ ≥1.7 μm) generate recollision electron wave packet energies sufficient (≥100 eV) to directly probe the ‘independent’ atomic cores in the molecule [31] , [36] , [38] . In this study, fixed-angle broadband laser-driven electron scattering (FABLES) is proposed as an alternative to fixed-energy, angle-swept LIED [36] . FABLES is analogous to white light interferometry in optics [39] , and this is the first experimental confirmation that broadband electron wave packet can be used for imaging. The main benefit of FABLES is a trivial retrieval of molecular structure via a simple Fourier transform (FT) with no theoretical fitting or modelling, for example, no a priori knowledge of laser ionization. Furthermore, the method ‘visualizes’ only bonds parallel to the laser polarization and has the potential for routine, real-time imaging in a pump-probe configuration. This unique aspect combined with molecular alignment is shown theoretically to offer a full molecular tomographic reconstruction. Advantages of FABLES The benefit of FABLES over LIED is the potential application for imaging large molecules. In FABLES, the relevant molecular interference fringes are visible and easily extracted from the measured DCS (see Supplementary Fig. 2 and Supplementary Discussion ). The terms contributing to the DCS in LIED and FABLES are similar to the CED data: each consists of a large incoherent atomic scattering term and a small-amplitude, structure-sensitive oscillation due to the molecular interference [3] , [36] . Therefore, the main challenge in extracting structural information from measured DCS consists of separating the usually weak interference term from the dominant atomic ones. In the N 2 and O 2 LIED experiment [36] , extracting the small (~15% of the atomic DCS) molecular interference term from the fixed-energy, angular-dependent molecular DCS required considerable theoretical effort due to the nontrivial angular dependence of atomic DCS. This is manageable for simple molecules, for example, diatomics, but extrapolation to larger systems is tenuous. Fortunately, two independent effects provide a much simpler alternative method, FABLES. First, the energy-dependent atomic DCS for backscattering geometry ( θ r =180°) shows only a simple smooth, Rutherford-like behaviour (see Supplementary Figs 2b and 3a,b ). In this case, the weaker oscillatory interference component is directly visible and thus easily rectifiable from the DCS. This behaviour is universal even for large molecules. Second, strong-field experimental and theoretical studies [31] , [40] , [41] , [42] have shown that the returning broadband wave packet (RWP) energy distribution is also a smooth continuous function, further facilitating extraction. 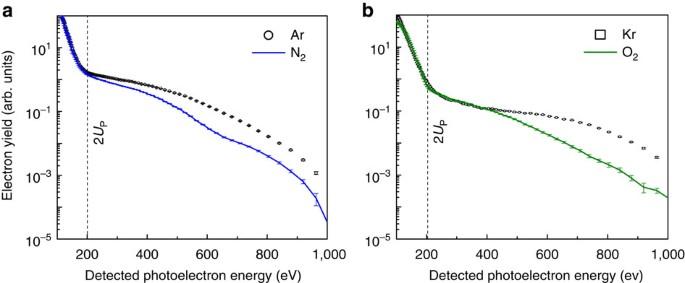Figure 1: High-resolution photoelectron energy distributions along the laser polarization. (a) Nitrogen and argon recorded at a wavelength of 2.0 μm and an intensity of 270 TW cm−2. The error bars indicate theN−1/2Poisson statistical fluctuations for each time bin,Nbeing the number of detected electrons in the bin. The vertical dashed line marks the 2UPenergy, electrons below this are direct. Above it, the long plateau corresponds to photoelectrons that are backscattered following ionization. The plateaus are a direct illustration of the broadband nature of the returning electron wave packet. (b) The oxygen and krypton distributions at a wavelength of 2.5 μm and an intensity of 130 TW cm−2. Experimental data and intramolecular interference fringes Figure 1 shows the backscattered photoelectron energy distributions for nitrogen and oxygen molecules measured in a time-of-flight spectrometer (see Methods) using 2–2.5 μm, 60 fs laser pulses at constant U P =100 eV. Each molecule is accompanied by its corresponding atomic partner with similar ionization potential (Ar/N 2 and Kr/O 2 ) to retrieve the RWP [43] . Given the small magnitude of the expected interference signal, the rescattered plateaus (energies greater than the dashed black lines) were recorded with 1–3% statistical fluctuations. For each atom–molecule pair, the spectra were normalized such that the direct electrons (<2 U P , below vertical dashed line) overlap. For both pairs, the direct electron distributions show remarkable agreement, confirming the assertion that in the strong field limit, the ionization rate and hence the electron wave packet spectral densities depend mainly on the value of the ionization potential [43] . Figure 1: High-resolution photoelectron energy distributions along the laser polarization. ( a ) Nitrogen and argon recorded at a wavelength of 2.0 μm and an intensity of 270 TW cm −2 . The error bars indicate the N −1/2 Poisson statistical fluctuations for each time bin, N being the number of detected electrons in the bin. The vertical dashed line marks the 2 U P energy, electrons below this are direct. Above it, the long plateau corresponds to photoelectrons that are backscattered following ionization. The plateaus are a direct illustration of the broadband nature of the returning electron wave packet. ( b ) The oxygen and krypton distributions at a wavelength of 2.5 μm and an intensity of 130 TW cm −2 . Full size image In contrast to the low-energy part (<2 U P ), the high-energy plateaus (2–10 U p ) of each atom–molecule pair exhibit clear differences. First, the atom’s plateau is enhanced compared with its molecular counterpart. In accordance to the quantitative rescattering theory [40] , the detected electron yield can be expressed as a product of electron’s RWP and the field-free DCS. In Supplementary Fig. 3a,b , it is shown that the backscattered, energy-dependent DCS for the two noble gases are approximately an order of magnitude larger than their molecular partner, confirming that for each pair the relative RWP amplitudes are approximately the same [43] . Second, a closer inspection of the Ar-N 2 plateaus ( Fig. 1a ) reveals a distinct modulation present in nitrogen but not in argon. As shown in the Supplement (see Supplementary Fig. 3a,b ), at high collision energies, electron-atom backscattering DCS is monotonically decaying and structureless. Consequently, the modulation must be attributed to the intramolecular term, which is produced by interfering backscattered waves emanating from each atomic core, analogous to the two-centre effect observed in high harmonic generation [44] , valence/core-shell photoionization spectrum [45] , [46] and ion impact electron ionization spectrum [47] from a diatomic molecule. Additional experimental confirmations were established at other driving laser wavelengths (see Supplementary Fig. 3c and Supplementary Discussion ). Thus, the N 2 structure is encoded in the interference patterns. On the other hand, the plateau of O 2 ( Fig. 1b ) reveals no modulation. Ionization-induced apparent alignment and collision geometry The difference between N 2 and O 2 is explained by examining the dependence of the ionization rate as a function of molecular orientation, as shown in the polar plots of Fig. 2 . In a linearly polarized field, nitrogen (oxygen) molecules ionize more readily on (off) the molecular axis. The net effect is that although both gases are randomly oriented in the interaction region, the detected signal mostly originates from molecules possessing the ‘optimal’ orientation for ionization, as illustrated in Fig. 2a,b . The resulting influence on the calculated DCS (see Methods for theoretical details) is shown in Fig. 2c,d . For reference, the corresponding incoherent atomic DCS for each molecule is also shown (dashed lines). For nitrogen, a clear (~±20%) modulation is observed, whereas for oxygen the modulation is <±3%, both results are consistent with the experiment. 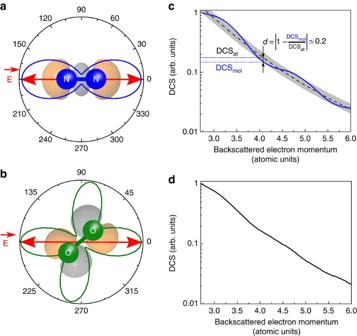Figure 2: Effect of the ionization rate as a function of molecular alignment angle on the elastic backscattering differential cross-sections. For a randomly distributed N2/O2gas, the ionization rate maximizes when the molecule is aligned so that the laser polarization axis is parallel to the lobes of the electron cloud of the highest-occupied molecular orbital (HOMO). The HOMOs of N2and O2have different symmetries,σandπ, respectively, which are depicted inaandbby the colour density plots, as well as their associated molecules in the ball-and-stick model. (a,c) The ionization rate (blue) of N2favors molecules that are aligned with respect to the laser polarization axis, which is the incident direction of the rescattered electrons. The resulting backscattering collision geometry for nitrogen is along the molecular axis. The calculated backscattering elastic DCS as a function of electron momentum for a randomly oriented gas with the ionization probability included (blue solid line). The featureless atomic term is also shown (black dashed line). The total DCS displays a clear oscillatory behaviour with a modulation depthd=±20%. The grey-shaded area indicates the modulation depth. (b,d) Same for oxygen except now that theπsymmetry of O2HOMO causes an off-axis collisional geometry, which results in a small modulation depth<±3% in the DCS, too small to be visible in the experiment. Figure 2: Effect of the ionization rate as a function of molecular alignment angle on the elastic backscattering differential cross-sections. For a randomly distributed N 2 /O 2 gas, the ionization rate maximizes when the molecule is aligned so that the laser polarization axis is parallel to the lobes of the electron cloud of the highest-occupied molecular orbital (HOMO). The HOMOs of N 2 and O 2 have different symmetries, σ and π , respectively, which are depicted in a and b by the colour density plots, as well as their associated molecules in the ball-and-stick model. ( a , c ) The ionization rate (blue) of N 2 favors molecules that are aligned with respect to the laser polarization axis, which is the incident direction of the rescattered electrons. The resulting backscattering collision geometry for nitrogen is along the molecular axis. The calculated backscattering elastic DCS as a function of electron momentum for a randomly oriented gas with the ionization probability included (blue solid line). The featureless atomic term is also shown (black dashed line). The total DCS displays a clear oscillatory behaviour with a modulation depth d =±20%. The grey-shaded area indicates the modulation depth. ( b , d ) Same for oxygen except now that the π symmetry of O 2 HOMO causes an off-axis collisional geometry, which results in a small modulation depth<±3% in the DCS, too small to be visible in the experiment. Full size image Structural retrieval To retrieve the structural information, we adopt the mature rectification-based analysis method of CED [3] . 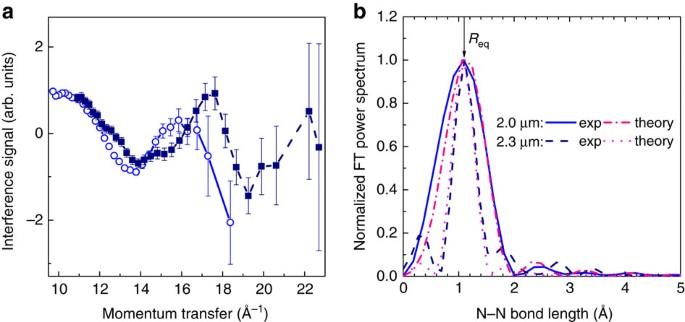Figure 3: FABLES-bond length retrieval and Fourier transform. (a) The intramolecular interference fringes extracted from the nitrogen plateau data at 2.0 μm (light blue open circles) and 2.3 μm (dark blue solid squares). The error bars represent the standard deviations of the two data sets, which are calculated from measurement errors of their corresponding photoelectron energy distribution by assuming that the theoretical atomic DCS is exact. (b) The mean internuclear distance function obtained by Fourier Transform of the data ina. The dash-dotted and dotted lines are the FT of the theoretical DCS spanning the same momentum transfer range as the experiments at 2.0 μm and 2.3 μm, respectively. The vertical arrow inbdenotes the known N2equilibrium distance,Req. Our retrieved bond lengths deviate fromReqby 0.01 Å. Figure 3a shows the intramolecular interference fringes extracted from the nitrogen distributions at 2.0 and 2.3 μm as a function of the momentum transfer | q |. Following CED’s inversion procedure, a Fourier transform extracts from the momentum-space interferogram the real-space structural information, as illustrated in the power spectra plotted in Fig. 3b . The internuclear distance functions retrieved from the experimental data peak at nearly the same position, 1.09 and 1.11 Å for 2.0 and 2.3 μm experiments, respectively. In comparison, the nitrogen equilibrium distance, R eq , is 1.10 Å. It is worth noting that as the electron return time varies with rescattering energies, for example, the RWP is chirped, the extracted distances here are the average length of the nitrogen bond over the temporal slit defined by the energy range used in the analysis (roughly a quarter of the 6–7 fs laser cycle). Also plotted in Fig. 3b is the FT result for the theoretical DCS, covering the same | q |-range as the 2.0-μm and 2.3-μm data, respectively. The agreement with the experiment is excellent. The | q | values used in this study are comparable to that achieved in a CED experiment. We emphasize that the FT power spectrum strength is strongly affected by the modulation depth in Figs. 2c and 3a . As seen in Fig. 3b , the FT width of the internuclear distance peak is determined by the range of momentum transfer | q |, that is, a larger | q | range results in a narrower peak in space. One technical challenge for applying FABLES to large molecules is maintaining a sufficiently large value of | q | over a broad range for resolving different bonds. In principle, longer wavelength drivers (>5 μm) can fulfil this requirement. Figure 3: FABLES-bond length retrieval and Fourier transform. ( a ) The intramolecular interference fringes extracted from the nitrogen plateau data at 2.0 μm (light blue open circles) and 2.3 μm (dark blue solid squares). The error bars represent the standard deviations of the two data sets, which are calculated from measurement errors of their corresponding photoelectron energy distribution by assuming that the theoretical atomic DCS is exact. ( b ) The mean internuclear distance function obtained by Fourier Transform of the data in a . The dash-dotted and dotted lines are the FT of the theoretical DCS spanning the same momentum transfer range as the experiments at 2.0 μm and 2.3 μm, respectively. The vertical arrow in b denotes the known N 2 equilibrium distance, R eq . Our retrieved bond lengths deviate from R eq by 0.01 Å. Full size image The above results establish FABLES as an alternative LIED-based imaging approach [36] . Although the experiments described here hinge upon the unique strong field ionization properties of nitrogen, FABLES does have the potential to be developed into a powerful ultrafast imaging tool when combined with molecular alignment. Larger molecules, possessing several interatomic distances, would require high degrees of alignment, in addition to mid-infrared FABLES pulses. In general, 3D alignment is necessary to reconstruct the stereo-structure of a molecule without a priori knowledge since the information obtained from randomly oriented molecules is restricted to the radial function [1] , [3] , [48] , that is, internuclear distances. Thus, by combining the 1D FABLES with 3D molecular alignment/orientation techniques [48] , [49] , [50] , 3D imaging can be conducted analogous to the computer-assisted tomographic scanning method, now widespread in medical imaging. In such an experiment, a polarization-controlled aligning pulse rotates the molecule with respect to the polarization axis of a FABLES probe pulse delayed by the rotational revival time. At each aligning angle a 1D spectrum with its FT is recorded, thus transforming FABLES into a 2D/3D molecular tomography. A second advantage of FABLES is its bond selectivity. As shown above and described further in the Supplement (see Supplementary Fig. 4 and Supplementary Discussion ), molecular bonds aligned parallel to the FABLES axis show a good modulation, whereas off-axis bonds do not. This could prove to be an important advantage, as it will allow one to only ‘see’ a desired molecular bond during the experiment. This visualization of isolated molecular bonds, combined with its inherently high temporal resolution, makes FABLES a very exciting technique for actually ‘watching’ chemical bonds form and break. Experimental setup The tunable light source (0.7–1.0 mJ, 60 fs, 2–2.3 μm) used in the experiment consists of an optical parametric amplifier (Topas-HE by LightConversion) pumped by a titanium:sapphire front end system (6.2 mJ, 50 fs, 0.8 μm, 1 kHz). The mid-infrared pulses were focused using a 100-mm focal length CaF 2 lens into a 22-cm field-free, time-of-flight electron spectrometer. A small, ±0.8° collection angle for increased angular resolution was obtained by placing a 6-mm diameter pinhole in front of the 40 mm diameter multichannel plate detector located at the end of the flight tube. The modulation depth of the interference term visible in the nitrogen plateau ( Fig. 1 ) is of the order of ±20%, spanning the energy range from 200 to 1,000 eV. To detect this oscillation, a time to digital converter with 250-ps time bins was used. For each gas target and each wavelength, ~10 7 laser shots were taken, assuring better than 3% statistical fluctuations across the entire plateau, as illustrated by the small error bars in Fig. 1 . In principle, the entire electron’s momentum distribution can also be taken using techniques such as velocity map imaging. However, these techniques are currently incapable for detecting electrons over a broad range extending into the kiloelectron volt region. Extraction of interference fringes We first follow the quantitative rescattering theory [40] to extract the collision-energy-dependent molecular DCS of nitrogen from the photoelectron energy distribution; the background signal, that is, atomic scattering DCS and electron RWP, is then removed, leaving only the oscillating interference fringes. The electron RWP distribution W (| k r |), defined as D ( k )/ σ ( k r ) in the quantitative rescattering theory, is obtained from the photoelectron spectrum of argon under identical laser conditions. W (| k r |) has been shown to follow a universal scaling law, independent of target species [31] , [51] . Here D ( k ) is the plateau electron spectrum, σ ( k r ) is the field-free elastic scattering DCS and k is the detached photoelectron momentum (for the relationship of k and k r , see ref. 36 ). Note that the measurement of photoelectron angular distribution of the companion atom for background removal is not necessary. In principle, due to the smoothness of the atomic scattering cross-sections and electron returning wave packet, the background signal has a trivial monotonic dependence on collision energy and therefore can be eliminated empirically, which is a common practice in CED [3] . Theoretical methods The method used to calculate the molecular scattering DCS is the well-documented independent atom model (IAM). In IAM, the molecule is modelled as a collection of non-interacting atoms located at { R i , i =1,…, N }, and the molecular scattering amplitude F ( E , Ω; Ω L ) is a coherent summation of atomic scattering amplitudes { f i , i =1,…, N }, where N is the total number of atoms in the molecule, q is the momentum transfer as defined in the main text, Ω L is the molecular alignment angle, and E and Ω are the scattering energy and angle, respectively. The DCS of diatomic molecules is written as, which reveals the important features of electron diffraction from a molecule. The first term on the right-hand side, dubbed atomic term, constitutes an incoherent sum of atomic diffracted waves originating at individual nuclei and carries no molecular structure information. Conversely, the second term, called the intramolecular interference term, depends upon internuclear separations R ij = R i − R j . More details about IAM and calculation of atomic scattering amplitudes f i have been discussed in our previous publications, see ref. 38 and the Supplementary Materials of refs 31 , 36 . In the current study, the orientation-dependent ionization rate Γ (Ω L ) functions as an actual alignment of the molecule, which is crucial to obtain a good contrast of the interference fringes. The molecular ionization rates of N 2 and O 2 are calculated based on the molecular Ammosov-Delone-Krainov theory [52] , and IAM-based molecular scattering DCS at different alignment angle Ω L are weighted by Γ ( Ω L ) to simulate the experimental results. How to cite this article: Xu, J. et al. Diffraction using laser-driven broadband electron wave packets. Nat. Commun. 5:4635 doi: 10.1038/ncomms5635 (2014).